The mechanism of caesium intercalation of graphene Properties of many layered materials, including copper- and iron-based superconductors, topological insulators, graphite and epitaxial graphene, can be manipulated by the inclusion of different atomic and molecular species between the layers via a process known as intercalation. For example, intercalation in graphite can lead to superconductivity and is crucial in the working cycle of modern batteries and supercapacitors. Intercalation involves complex diffusion processes along and across the layers; however, the microscopic mechanisms and dynamics of these processes are not well understood. Here we report on a novel mechanism for intercalation and entrapment of alkali atoms under epitaxial graphene. We find that the intercalation is adjusted by the van der Waals interaction, with the dynamics governed by defects anchored to graphene wrinkles. Our findings are relevant for the future design and application of graphene-based nano-structures. Similar mechanisms can also have a role for intercalation of layered materials. Rapid advance in epitaxial growth has resulted in uniform large-area high-quality epitaxial graphene (e-Gr) [1] , [2] , [3] , a prerequisite for future applications of graphene [4] , [5] . In search for novel properties, e-Gr systems are often modified with different atoms or molecules intercalated between graphene and its support—for example, to decouple graphene from its substrate by reducing the bonding interaction [6] , [7] . One important aspect of intercalation is chemical doping of graphene sheets [8] , an effect similar to electric field doping in field-effect graphene transistors [9] . Compared with field-induced doping, chemical doping has the additional options to open a band gap at the Dirac point [10] or even shift the the Fermi level up to the extended π* band van Hove singularity of graphene [11] . The diversity and sensitivity of the physical and chemical properties of e-Gr [8] , graphite [12] , [13] and other layered systems [14] with respect to intercalation of charge-donating species are directly related to prominent effects, such as superconductivity in graphite [15] , [16] and the uncharted one in graphene [17] , [18] . From the view point of chemical kinetics, understanding the penetration and diffusion of ions under graphene sheets in atomistic detail is of fundamental importance for the design of novel batteries and supercapacitors [19] . There are other potentially useful properties associated with the intercalation of e-Gr systems. For instance, it was demonstrated that by precise control of the intercalation interface, laterally well-defined mesoscopic regions of n - and p -doped graphene—that is, p–n graphene junctions, can be formed [20] . It was also demonstrated that it is possible to form well-defined ferromagnetic nano-islands under e-Gr [21] . Therefore, it is important to understand in detail how the properties of chemically modified graphene depend on its chemical environment. For example, for spintronic applications, on the one hand, intercalation of ferromagnetic 3d metals such as Co (ref. 22 ) or Ni (refs 21 , 23 ) is explored; however, it results in a strong chemical interaction between the metal d-orbitals and π-bands of graphene. On the other hand, a more promising approach to design magnetic properties of graphene by using its almost unperturbed π-bands is the intercalation of a wider class of systems of the same nature—such as, alkali metals, alkaline earth metals or lanthanides (for example, Nd or Eu that contain 4f and 6s electrons) [24] . Graphene on Ir(111), e-Gr/Ir, is recognized for its unique structural quality [25] and weak bonding to the substrate [26] that results in an electronic structure resembling that of freestanding graphene [27] , [28] . Despite macroscopic uniformity, it was shown that different metals and molecules can be successfully intercalated between graphene and iridium [22] , [23] , [24] , [29] , [30] , [31] , [32] , [33] , [34] , [35] . These findings not only call for an explanation on how the intercalation can occur through an apparently perfect graphene membrane but also for the mechanism driving the intercalation. Here we characterize the process of adsorption and intercalation of Cs in microscopic detail by utilizing in situ low-energy electron microscopy (LEEM), scanning tunnelling microscopy (STM), low-energy electron diffraction (LEED), angle-resolved photoemission spectroscopy (ARPES) and density functional theory (DFT) calculations. For comparison, we characterize also the intercalation of Li, which has a much smaller ionic radius than Cs. We describe the energetics and the novel mechanisms that explain the kinetics of intercalation and entrapment of alkali atoms under epitaxial graphene. We find that these processes are regulated by the vdW interaction, with defects at graphene wrinkles acting as penetration sites for alkali atoms. The reported mechanism may be specific to the particular system studied. Nevertheless, we believe that our study represents a very important and necessary step in gaining a fundamental knowledge on the s–π interactions and the intercalation process itself. This information can be further used to unveil the properties of more complicated intercalated systems—for example, where additional complex spin-dependent interactions take place. Characterization of the adatom and intercalated phases The experiments presented below indicate the formation of two phases upon Cs deposition on e-Gr/Ir. After the initial dilute phase on graphene, the α-phase, reaches its maximum density at about 0.06 monolayer (ML), additionally deposited Cs is intercalated and forms the γ-phase as a (2 × 2) structure. Upon further deposition, the area fraction of the γ-phase increases at the expense of the area fraction of the α phase. Once the entire sample is transformed to the γ phase, it further becomes denser through the applied Cs pressure until the saturation density is eventually reached, when the γ-phase has the ( × )R30° structure relative to Ir(111) at a coverage taken as a definition of 1 ML of Cs. 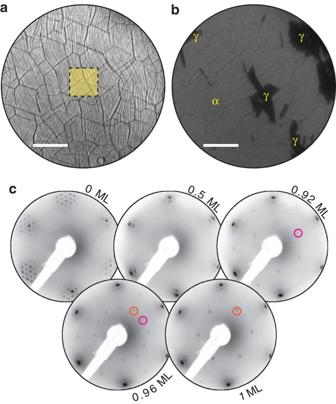Figure 1: LEEM and LEED characterization. (a) LEEM topograph of an uniform e-Gr ML on Ir(111) showing characteristic surface features: graphene wrinkles and substrate steps. The yellow square indicates the area analysed for the dynamics of intercalation (cf.Fig. 5). (b) Same area as inabut after deposition of 0.2 ML of Cs. A moderate decrease (α-phase, marked as α) and a strong decrease (γ-phase, marked as γ) in reflectivity are visible. Scale bars ina,bcorrespond to 3 μm. (c) LEED patterns of structures obtained for various amounts of deposited Cs (indicated for each pattern). The 0-ML pattern was recorded at 117 eV and all remaining patterns at 130.5 eV electron energy. Magenta circles indicate a (2 × 2) structure relative to e-Gr, whereas orange circles indicate a (×)R30° structure relative to Ir. Figure 1 shows the fingerprints of structures being formed in the process of intercalation. The corresponding LEEM image of the initial e-Gr/Ir surface ( Fig. 1a ) reveals several structural features. Thick dark lines are wrinkles—graphene areas delaminated from the substrate—a signature of strain release in graphene [36] , [37] . In addition, steps of the Ir(111) substrate are resolved, which wiggle mostly vertically as well as diagonally (several straight glide steps) through the image. The LEEM images were recorded for various amounts of deposited Cs, up to 1 ML. Figure 1b shows a LEEM micrograph of the surface after deposition of 0.2 ML of Cs. Dark regions with sharp boundaries are visible and attributed to the γ-phase. The remaining homogeneous surface contrast is attributed to the α-phase. For more details on LEEM characterization see Supplementary Note 1 and Supplementary Movie 1 . In addition to LEEM imaging at fixed electron energy, we also performed the IV -LEEM measurements before and after deposition of 0.2 ML of Cs. The characteristic reflectivity curves from pristine e-Gr/Ir, the α-phase and the γ-phase areas are shown in Supplementary Fig. S1 . The origin of apparent contrast differences in Fig. 1a,b is clearly visible in the reflectivity curves at the imaging energy of 1.5 eV. The γ-phase reflectivity shows a dip with a minimum close to that energy, which is a clear indication of the formation of a new dense layer [38] . Figure 1: LEEM and LEED characterization. ( a ) LEEM topograph of an uniform e-Gr ML on Ir(111) showing characteristic surface features: graphene wrinkles and substrate steps. The yellow square indicates the area analysed for the dynamics of intercalation (cf. Fig. 5 ). ( b ) Same area as in a but after deposition of 0.2 ML of Cs. A moderate decrease (α-phase, marked as α) and a strong decrease (γ-phase, marked as γ) in reflectivity are visible. Scale bars in a , b correspond to 3 μm. ( c ) LEED patterns of structures obtained for various amounts of deposited Cs (indicated for each pattern). The 0-ML pattern was recorded at 117 eV and all remaining patterns at 130.5 eV electron energy. Magenta circles indicate a (2 × 2) structure relative to e-Gr, whereas orange circles indicate a ( × )R30° structure relative to Ir. Full size image Figure 1c shows the emerging structures observed using LEED, recorded at room temperature. The diffraction spots of e-Gr/Ir before deposition reveal the characteristic moiré pattern of uniformly aligned graphene. For coverages below 0.9 ML, no clear Cs superstructure is observed in LEED (cf. 0.5 ML). Apparently, at room temperature intercalation islands of finite size do not exhibit a stable crystal structure. This was further corroborated by a micro-LEED imaging in the LEEM setup (not shown). Only at high coverages of ~0.9 ML and above, or at low temperatures, well-defined superstructures of intercalated Cs are observed. In the range from 0.9 to 1 ML of Cs, we find in LEED: a (2 × 2) structure relative to e-Gr (for 0.92 ML), a mixture of a (2 × 2) relative to e-Gr and a ( × )R30° structure relative to Ir (for 0.96 ML) and finally for 1 ML a ( × )R30° pattern relative to Ir. In addition, the relevant superstructures are presented in Supplementary Table S1 . The electronic structure of e-Gr/Ir in Fig. 2a is characterized by a sharp Dirac cone, exhibiting slight p -doping of graphene, consistent with previous experiments [27] , [28] . The deposition of Cs leads to the following modifications of the ARPES spectra: for low Cs coverage, of up to ~0.06 ML, the Dirac cone of slightly p -doped e-Gr/Ir shifts progressively to higher binding energies as the Cs coverage is increased. The Dirac point shifts down to 0.2 eV below the Fermi level, making graphene slightly n -doped. From the ARPES spectra, we obtain that the maximum electron doping in the α-phase is n ≈4 × 10 12 cm −2 corresponding to a charge transfer of 0.11 electrons from each Cs atom in the α-phase to graphene (see Supplementary Fig. S2 ). For more than ~0.06 ML, an additional Dirac cone appears at higher binding energy because of phase separation; Fig. 2b corresponds to 0.5 ML of Cs and it shows two Dirac cones, light and heavily electron-doped, corresponding to the α-phase and the γ-phase, respectively. The α-phase cone decreases in intensity and completely disappears above ~0.9 ML of Cs and only the γ-phase cone remains visible. Once the entire sample is covered by the γ-phase, additional deposition from 0.9 to 1 ML ( Fig. 2c ) increases its density, consistent with the evolution of the LEED patterns and the additional shift of the Dirac point (see Supplementary Fig. S3 and Supplementary Note 2 ). The maximum doping of n ≈1 × 10 14 cm −2 implies a charge transfer of 0.20 electrons per Cs atom to graphene. 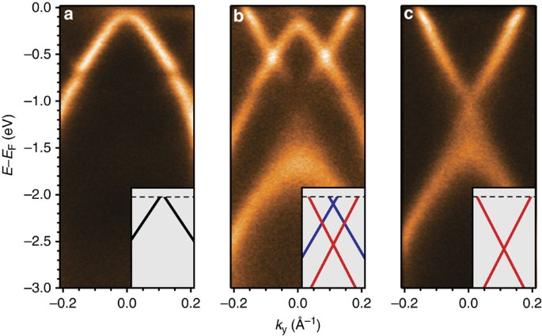Figure 2: ARPES characterization. ARPES maps (vertical axis: binding energyE−EFreferenced to the Fermi levelEF, horizontal axis: wave vectorky) taken across the K point of graphene for different amounts of deposited Cs: (a) pristine graphene, (b) 0.5 ML and (c) 1 ML of Cs. Insets ina–cschematically indicate Dirac cones visible in ARPES maps, corresponding to pristine (black), light (blue) and heavily (red) electron-doped Dirac cones. Figure 2: ARPES characterization. ARPES maps (vertical axis: binding energy E − E F referenced to the Fermi level E F , horizontal axis: wave vector k y ) taken across the K point of graphene for different amounts of deposited Cs: ( a ) pristine graphene, ( b ) 0.5 ML and ( c ) 1 ML of Cs. Insets in a – c schematically indicate Dirac cones visible in ARPES maps, corresponding to pristine (black), light (blue) and heavily (red) electron-doped Dirac cones. Full size image Additional insight comes from STM. After deposition of 0.5 ML Cs at room temperature and cooling the sample to 6 K prior to STM measurements to enable stable imaging, two characteristic areas can be distinguished in the topographs. As shown in Fig. 3a , we identify the area with disordered bright protrusions corresponding to Cs adatoms as the α-phase. The concentration of adatoms varies slightly over the sample surface with the maximum corresponding to hexagonally arranged atoms at a nearest neighbour distance of 1.86±0.01 nm—that is, 0.063 ML. The flat area of Fig. 3a is apparently 0.4 nm higher than its surrounding, indicative for the presence of an additional dense layer, which we attribute to the γ-phase. Finally, note straight and thin channels in the intercalation mesa, which we relate to the inhomogeneous binding of graphene to the substrate-marking areas with comparatively high delamination energy [24] . A more detailed STM characterization of the γ-phase is possible through high-resolution STM imaging. The STM topographs in Fig. 3b,c show atomic resolution obtained while scanning over two different intercalated areas. In both images, one can resolve the graphene unit cell as well as a weak moiré superstructure. This is also visible in the Fourier transforms of the STM images shown in Fig. 3b,c insets. A closer inspection of the images and their Fourier transforms enables an identification of the two different underlying Cs superstructures: the (2 × 2) structure relative to graphene in Fig. 3b and the ( × )R30° structure relative to iridium in Fig. 3c . The STM findings are thus fully in agreement with LEED characterization. 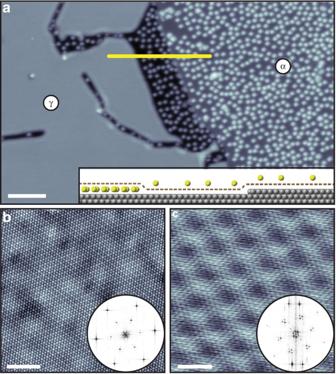Figure 3: STM characterization. (a) An STM topograph showing two characteristic areas found after the deposition of 0.5 ML of Cs: the adatom α-phase (marked as α) and the intercalated γ-phase (marked as γ). The inset shows a schematic illustration of the topographic profile across different regions of the STM image indicated by a yellow horizontal line. White scale bar corresponds to 10 nm. (b,c) High-resolution STM topographs of two different structures revealed in the γ-phase areas: (2 × 2) relative to graphene inband (×)R30° relative to Ir inc. The circular insets inb,cshow the corresponding Fourier transforms, the scale bars correspond to 3 nm. All images were recorded at 6 K. Figure 3: STM characterization. ( a ) An STM topograph showing two characteristic areas found after the deposition of 0.5 ML of Cs: the adatom α-phase (marked as α) and the intercalated γ-phase (marked as γ). The inset shows a schematic illustration of the topographic profile across different regions of the STM image indicated by a yellow horizontal line. White scale bar corresponds to 10 nm. ( b , c ) High-resolution STM topographs of two different structures revealed in the γ-phase areas: (2 × 2) relative to graphene in b and ( × )R30° relative to Ir in c . The circular insets in b , c show the corresponding Fourier transforms, the scale bars correspond to 3 nm. All images were recorded at 6 K. Full size image DFT calculations The main result of our DFT calculations is shown in Fig. 4a , where the binding energies for different Cs coverages corresponding to the adatom and intercalated phases are plotted. Calculations with the vdW interaction included show a clear crossover between the adatom and intercalated phases for dilute and dense concentrations, respectively. For considered Cs concentrations, the charge transfer in the adatom and the intercalated phase is visualized in Fig. 4b . Looking at the charge transfer alone, the main difference between the intercalated and the adatom structure comes from the much larger amplitudes of charge rearrangement in the intercalated system. There, the Cs atom causes a large redistribution of charge on both, the Ir surface and the graphene (lower row of Fig. 4b ), mimicking the electrostatic glue for floating n -doped graphene. In contrast, in the adatom case most of the charge rearrangement takes place on the graphene sheet close to Cs (upper row of Fig. 4b ). In order to determine the importance of the vdW interaction, in Fig. 4a we also present the results obtained using a semi-local functional, which does not contain the vdW correlation effects. This functional fails to correctly describe the experimental observations (see below and also Supplementary Figs S4, S5 and Supplementary Note 3 ). 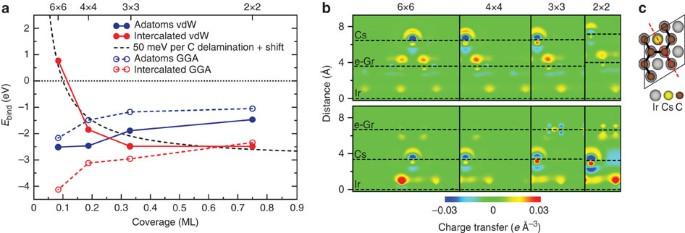Figure 4: Binding energies and charge transfer calculations. (a) Binding energies (Ebind) as a function of Cs coverage in ML for the intercalated and the adatom phase. The plotted values are given per unit cell used in the calculations and referenced to the corresponding pristine e-Gr/Ir system plus a free Cs atom. The open symbols and dashed lines show the results obtained using the GGA functional, whereas the full symbols and full lines are obtained with the inclusion of the non-local vdW correlation. The dashed black line is a guide to the eye simulating a 50-meV delamination energy per C-atom plus a constant offset. (b) Charge transfer (colour-coded in units of electrons per Å3) in the adatom phase (upper row) and in the intercalated phase (lower row). The corresponding Cs concentrations are marked on top of the panel. Black-dashed lines indicate the positions of Ir, e-Gr and Cs layers. (c) A model indicating the position of a geometric plane (dashed red) across which the charge transfer inbis plotted. Figure 4: Binding energies and charge transfer calculations. ( a ) Binding energies ( E bind ) as a function of Cs coverage in ML for the intercalated and the adatom phase. The plotted values are given per unit cell used in the calculations and referenced to the corresponding pristine e-Gr/Ir system plus a free Cs atom. The open symbols and dashed lines show the results obtained using the GGA functional, whereas the full symbols and full lines are obtained with the inclusion of the non-local vdW correlation. The dashed black line is a guide to the eye simulating a 50-meV delamination energy per C-atom plus a constant offset. ( b ) Charge transfer (colour-coded in units of electrons per Å 3 ) in the adatom phase (upper row) and in the intercalated phase (lower row). The corresponding Cs concentrations are marked on top of the panel. Black-dashed lines indicate the positions of Ir, e-Gr and Cs layers. ( c ) A model indicating the position of a geometric plane (dashed red) across which the charge transfer in b is plotted. Full size image Intercalation and de-intercalation dynamics In addition to the phases described above, LEEM sequences taken during Cs deposition and desorption provide information on the kinetics of these processes (see Supplementary Notes 1, 4 and also Supplementary Movies 1, 2 ). The analysis of such sequences shows that the growth of the γ-phase is discontinuous, composed of sudden and rapid advancements, followed by extended periods of stagnation. This is visualized in Fig. 5 where snapshots of the same sample area at the indicated incremental times are displayed. An area of pristine e-Gr/Ir is shown in Fig. 5a . In Fig. 5b , the same area is shown but with the network of wrinkles (full lines) and steps (dotted lines). They divide the surface into an assembly of small tetragonal micro-tiles. We find that these features are essential for the evolution of the intercalated phase. In particular, the γ-phase always forms next to wrinkles, typically at crossing points of wrinkles. Virtually at any time, all boundaries of such intercalated islands are identified as wrinkles or surface steps ( Fig. 5c–i ). Hence, their expansion can be described as tiling. For the characteristic surface area studied in our work, the density of wrinkle- and step-line substructures differed almost by an order of magnitude, 1 μm −1 for wrinkles and 7 μm −1 for steps. Thus, once the intercalation island has nucleated, its discontinuity of expansion depends more strongly on the denser network of Ir-steps. They have the role of a kinetic barrier for diffusion of intercalated Cs atoms. An example of a tiling step is highlighted in panels 5h and 5i of Fig. 5 where an arrow points to an empty and a filled tile, respectively. 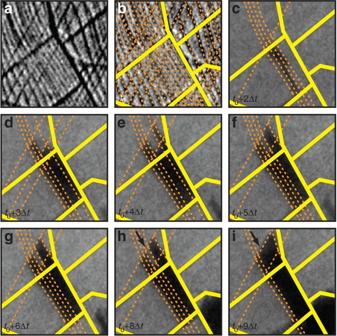Figure 5: Dynamics of intercalation. Series of (2.52 × 2.52) μm2LEEM frames showing the same surface area (a,b) before any Cs deposition and (c–i) after the appearance of the dark intercalated Cs islands. Snapshots were imaged at the indicated time intervals (Δt=72 s) with respect tot0, the reference time when imageawas taken. Inb, the entire network of wrinkles and steps is highlighted by full and dotted lines, respectively. Inc–i, only wrinkles and relevant steps are highlighted. In the last two panels, an arrow indicates an empty (h) and a filled tile (i). Figure 5: Dynamics of intercalation. Series of (2.52 × 2.52) μm 2 LEEM frames showing the same surface area ( a , b ) before any Cs deposition and ( c – i ) after the appearance of the dark intercalated Cs islands. Snapshots were imaged at the indicated time intervals (Δ t =72 s) with respect to t 0 , the reference time when image a was taken. In b , the entire network of wrinkles and steps is highlighted by full and dotted lines, respectively. In c – i , only wrinkles and relevant steps are highlighted. In the last two panels, an arrow indicates an empty ( h ) and a filled tile ( i ). Full size image As intercalated islands nucleate at crossing points of wrinkles, we assume that the entrance points for Cs atoms to pass under graphene are nano-scale cracks located at these crossing points, either as pre-existing defects that pin the wrinkles—that is, their ends or crossings—or as cracks that form during wrinkles formation because of extensive local forces. As a wrinkle is a three-dimensional (3D) feature, in LEEM it scatters electrons strongly and with poor coherence. This contributes to lowering the resolution and prevents to resolve structural inhomogeneities with LEEM. Our STM characterization of wrinkles of e-Gr/Ir in Fig. 6 enables more insight than LEEM. The widths (10–50 nm) and heights (1–5 nm) of different wrinkles vary. Most of the wrinkles orient independently across terraces and step edges, whereas some of them are pinned near to/at the step edges. Individual wrinkles can slightly change their direction and sometimes also width or height (cf. Fig. 6a ). In contrast to the homogeneous parts, the wrinkle crossing shown in Fig. 6b depicts a highly inhomogeneous structure. Although it is not possible to resolve cracks in such crumpled regions, their crumpling is consistent with being the entry areas for Cs atoms. Less extensive defects have already been characterized by STM in epitaxial graphene samples. Small graphene rotations within the sheet resulted in an array of heptagon–pentagon pairs [39] and larger rotations in nanometer-wide grain boundaries [40] . Moreover, it was proposed that a vacancy defect greater than four missing carbon atoms on a graphite surface is needed to allow Cs intercalation to the subsurface layers [41] . Although our LEED data indicate uniform graphene, small rotations (for example, below 1°) and the existence of heptagon–pentagon pairs cannot be entirely excluded. However, the LEEM and STM data indicate that highly defective areas at wrinkle crossings enable the transport of atoms across graphene layers. The role of these entry cracks is additionally described in the following desorption experiment. 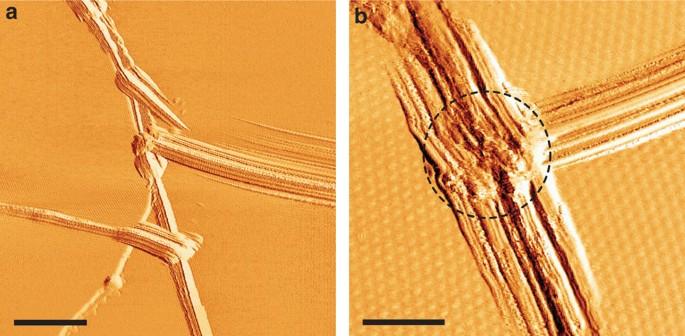Figure 6: STM characterization of wrinkles. (a) A large-scale STM topograph showing several wrinkles. Scale bar corresponds to 60 nm. (b) Area showing a crossing of two wrinkles. Scale bar corresponds to 15 nm. The characteristic moiré structure of graphene is visible in the areas around wrinkles. The crossing area highlighted by the dotted circle appears as a highly crumpled structure. Figure 6: STM characterization of wrinkles. ( a ) A large-scale STM topograph showing several wrinkles. Scale bar corresponds to 60 nm. ( b ) Area showing a crossing of two wrinkles. Scale bar corresponds to 15 nm. The characteristic moiré structure of graphene is visible in the areas around wrinkles. The crossing area highlighted by the dotted circle appears as a highly crumpled structure. 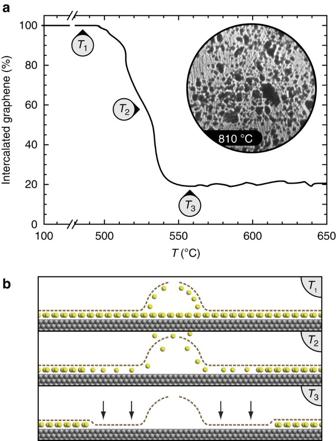Figure 7: Desorption of intercalated phase. (a) Black curve represents the γ-phase LEEM contrast as a function of the sample temperature, extracted by area integration from a LEEM movie. The inset shows the final movie frame with well-defined trapped intercalation islands (image diameter is 14 μm). (b) Schematic sketch of the system structures at various temperatures: right before desorption starts (T1), during Cs desorption (T2) and after desorption is suppressed by relamination of graphene areas (T3), as indicated by arrows. Full size image Figure 7a shows the analysis of the γ-phase LEEM contrast of the sample that was fully intercalated and then heated up to 810 °C. The entire desorption dynamics takes place in a narrow temperature range (500–550 °C), where 80% of the γ-phase contrast is lost and replaced by the contrast equivalent to pristine e-Gr/Ir. However, the remaining 20% of the γ-phase area does not vanish even at the highest recorded temperature; the characteristic LEEM topograph (inset of Fig. 7a ) shows well-defined dark pockets of the γ-phase. We interpret the desorption dynamics and its interruption as sketched in Fig. 7b . At about 500 °C, desorption takes place, by the principle of micro-reversibility, through the same channels that enabled intercalation—cracks in graphene associated with wrinkles. When the Cs concentration falls below a critical value, graphene will relaminate to Ir (cf. arrows in Fig. 7b lowermost panel). This will take place first in the surroundings of the entry/exit spots where the Cs has already been lost. Once an exit spot is surrounded entirely by relaminated e-Gr, no more desorption takes place through this spot. Eventually, very stable Cs pockets are trapped through the vdW adhesion of e-Gr to Ir(111). Figure 7: Desorption of intercalated phase. ( a ) Black curve represents the γ-phase LEEM contrast as a function of the sample temperature, extracted by area integration from a LEEM movie. The inset shows the final movie frame with well-defined trapped intercalation islands (image diameter is 14 μm). ( b ) Schematic sketch of the system structures at various temperatures: right before desorption starts ( T 1 ), during Cs desorption ( T 2 ) and after desorption is suppressed by relamination of graphene areas ( T 3 ), as indicated by arrows. Full size image Li intercalation To make our study more comprehensive, we have characterized also the intercalation of Li, which is on the opposite side of the alkali metals group. Details are presented in Supplementary Fig. S6 and Supplementary Note 5 . Our vdW density functional (vdW-DF) calculations show that intercalation is energetically more favourable even for the diluted Li structure. This is confirmed by our ARPES data (cf. Supplementary Fig. S7 ), which indicate the absence of phase separation as observed for Cs. Homogeneous chemical doping uniformly increases as Li is dosed and reaches its maximum when a (1 × 1) structure relative to Ir is formed. This is possible because Li, because of its small size, does not have to lift off graphene notably and pay much for delamination energy in order to form intercalated structures. Thereby, it can intercalate at any density with much smaller cost of graphene partial delamination. In the same manner, annealing of a Li-intercalated sample results in gradual and complete Li removal, indicating that no relamination effects take place. The observed kinetics of the system allows us to consider the mechanism of the intercalation. First, in the α-phase the binding of Cs adatoms to graphene originates mainly from the partial delocalization of the Cs s-electrons within graphene. However, the smaller the distance between the adatoms gets, the larger is the Coulomb repulsion penalty. Therefore, the binding energy decreases with increasing Cs coverage as shown by the blue data points in Fig. 4a ; the repulsive adatom–adatom interaction creates a two-dimensional (2D) pressure that increases with Cs coverage. The system relieves this pressure by emptying the adatom phase through intercalation. This is the driving force for intercalation, which takes place through entry cracks at wrinkle crossings. Initial intercalation is, however, prevented because of the energy cost of graphene delamination from its substrate, about 50 meV per C-atom [26] . The black-dashed line in Fig. 4a shows a fit to this value. As this value is fixed per unit area, intercalation is only favourable if a dense Cs-phase forms, where the delamination energy cost is shared among many Cs atoms in the same small area. As the full lines in Fig. 4 indicate for a (3 × 3) and a denser structure, intercalation is favoured over an adatom phase of the same density. The additional screening provided by the close proximity of the metallic substrate in the intercalated phase lowers the Coulomb repulsion penalty for delocalization and the corresponding energy gain overcompensates the energy cost of graphene delamination. Experimentally, at the coverage corresponding to a (3 × 3) structure, phase separation of the system into an even denser intercalation γ-phase and a dilute adatom α-phase is observed, consistent with the coverage dependence of the two phases as shown in Fig. 4a . In the calculations where the vdW interaction is neglected, graphene is essentially not bound to Ir(111). Thus, in such an inadequate picture no energetic penalty has to be paid for delamination; hence, the intercalated phase is always preferred [42] . Although the vdW interaction is perceived as a weak dispersive force with only minor effects in processes on surfaces dominated by chemical bonds—for example, in catalysis—the vdW binding is quite generic. This is best comprehended through the binding effect that scales with the interacting surface: it is rather small for small molecules; however, as a flat molecule increases in surface, the total amount of the vdW force adds up. A good example is the relatively large phthalocyanine molecule [43] , and the extreme limit is found in epitaxial growth of graphene on surfaces. Moreover, if the bonding of a large surface area of graphene competes with a more localized and a rather strong chemical interaction—such as Cs intercalation—then both energy scales may become comparable. In this case, the semi-local DFT calculations may even fail qualitatively in predicting surface structure. Without the vdW interaction included, intercalation is always preferred because of the better screening of Cs ions close to the Ir(111) substrate, even for dilute structures, contrary to the observation. This finding highlights the importance of the vdW interactions when modelling and understanding the intercalation/desorption process and points to the importance of the delamination/relamination energy in the process of transport of alkali atoms below graphene. Our findings are important for understanding the mechanism of intercalation in layered systems where binding across the layers is determined by the vdW interaction. The process of intercalation is the result of a complex interplay of the adsorbed and intercalated phases: the intercalation is triggered by the concentration of Cs that is large enough to overcome the vdW binding of graphene to Ir. The precise energy threshold for this process is determined by overcoming of the vdW binding of graphene to Ir through the binding provided by the intercalated Cs atom. The significance of the vdW energy parameter is much lower for Li, which upon intercalation does not significantly change the separation between graphene and Ir and thus can also form a dilute intercalation phase. At the nano-scale, the process of nucleation of the intercalation phase growth is guided by well-located structural features—that is, nano-cracks at wrinkles crossings. The substrate steps are kinetic barriers for the expansion of the intercalated layer. The intercalation layer binds the floating graphene on the metal surface by electrostatic forces. Finally, the vdW binding of graphene to the substrate is responsible for the entrapment of isolated islands of intercalated Cs atoms, which are chemically protected by graphene and thermally stable up to very high temperatures. Graphene preparation Ir(111) single crystals of the same type were used in all setups (99.99% purity and orientation accuracy better than 0.1°). The substrate was cleaned by standard techniques of ion sputtering, oxygen firing and annealing [28] and e-Gr was synthesized by a combination of temperature-programmed growth and chemical vapour deposition procedures [25] . This yields high-quality e-Gr of uniform orientation as was confirmed after each preparation by LEED. In ARPES setups, graphene quality was additionally verified by spectral width (sharpness) of the Dirac cone bands. The sample was always prepared in situ in ultra-high vacuum under the base pressure better than 5 × 10 −8 (ARPES) and 5 × 10 −9 (LEEM and STM) Pa. Alkali metal deposition and desorption Cs and Li were deposited by using commercially available alkali metal dispensers (SAES Getters) with the typical flux values of ~10 15 m −2 s −1 . During Cs deposition, the sample was kept at constant temperature: 300 K in ARPES and STM setups and 340 K in LEEM setup. During Li deposition, the sample was kept at 300 K. In Cs desorption experiments, the LEEM data were recorded at an approximately constant heating rate of 4 K s −1 in the overall temperature range between 80 and 810 °C. Li desorption was performed by annealing the sample in several steps up to the maximum temperature of 600 °C with the ARPES data being recorded after each step. LEEM Measurements were carried out in a commercial Elmitec LEEM III system equipped with an energy analyser, installed at beamline U5UA at NSLS synchrotron. Data were recorded at 340 K (except for Fig. 7a ), with LEEM system operating in bright-field mode. Imaging electron energy was fixed to 1.5 eV (Cs deposition) or 2.4 eV (Cs desorption), whereas the focus of the microscope was adjusted as required in order to optimize the visibility of emerging structures. Spatial resolution of the microscope was ~10 nm. ARPES Experiments were performed at the U13UB beamline at NSLS synchrotron and in ARPES-dedicated setup in Zagreb. At U13UB, 23.4-eV p-polarized light was used for excitation and spectra were recorded at 300 K with Scienta SES2002 electron energy analyser (10 meV energy and 0.14° angular resolution) in the direction perpendicular to ΓK ( Fig. 2 , Supplementary Figs S3, S6 ). The spot size on the sample was 0.1 × 0.1 mm 2 . In Zagreb, a helium-discharge lamp provided photons of energy of 21.2 eV and of mixed polarization. Data were recorded with Scienta SES100 electron energy analyser (25 meV total energy resolution and 0.2° angular resolution) at 300 K in the direction parallel to ΓK ( Supplementary Fig. S2 ). The spot diameter on the sample in this setup was ~2 mm. STM STM measurements on the intercalated system were performed at low-temperature in Cologne (CreaTec LT-STM). The data were collected at 6 K; the STM tip was virtually grounded and the sample was put to a bias voltage. The data recorded in this setup are presented in Fig. 3a (1 V, 10 pA), Fig. 3b (120 mV, 300 pA), Fig. 3c (40 mV, 300 pA) and Supplementary Fig. S2b (1.07 V, 30 pA). The STM characterization of wrinkles was performed in Zagreb (SPECS Aarhus STM). The data were collected at room temperature, with the STM tip grounded and the sample put to a bias voltage. In STM experiments, wrinkles are sensitive to interactions with the STM tip—that is, tip shape and tunnelling parameters. The data recorded in this setup are presented in Fig. 6a (780 mV, 750 pA) and Fig. 6b (150 mV, 240 pA). STM data analysis was performed in the WSxM software [44] . DFT calculations DFT calculations were performed with the VASP code [45] and the PAW implementation [46] . The plane wave energy cutoff of 440 eV and a 15 × 15 × 1 k -point grid were used. The Ir substrate was simulated with a slab consisting of five layers of iridium. A vacuum of 20 Å was provided in the z -direction separating the periodic slab images. The ionic positions were relaxed until forces were below 0.01 eV Å −1 . The self-consistently implemented vdW-DF [46] , [47] was used with opt-B88 as exchange part [48] . In the experiments, the e-Gr layer on Ir(111) forms an ~(10 × 10)/(9 × 9) structure [26] . In the calculations, we have modified the Ir lattice constant to make commensurate structures. The results are in good agreement with large supercell calculations [49] . (2 × 2), (3 × 3), (4 × 4) and (6 × 6) in-plane unit cells of graphene were used to calculate the corresponding Cs-induced superstructures, whereas (1 × 1) and (4 × 4) in-plane unit cells were used in the case of Li. All energy curves are calculated for the structures relaxed with the vdW-DF functional—that is, both generalized gradient approximation (GGA) [50] , and vdW-DF calculations are performed for the same geometry of the system. For testing purposes, we relaxed systems containing Cs atoms with the vdW-DF and GGA functionals. The geometries obtained are practically identical. This is not the case for the pristine e-Gr/Ir system. By using GGA virtually no graphene binding results, whereas vdW-DF yields a binding distance of 3.52 Å for a commensurate cell. Charge density differences and non-local energy contributions were obtained by making differences between the system and the system parts, that is Ir slab, graphene sheet and a Cs atom—calculated at coordinates they have in the relaxed system. Real space distribution of the non-local binding energy density, as defined in Caciuc et al. [51] was obtained with the JuNoLo code [51] , [52] , [53] . How to cite this article: Petrović, M. et al. The mechanism of caesium intercalation of graphene. Nat. Commun. 4:2772 doi: 10.1038/ncomms3772 (2013).